Probing the crystallographic orientation of two-dimensional atomic crystals with supramolecular self-assembly 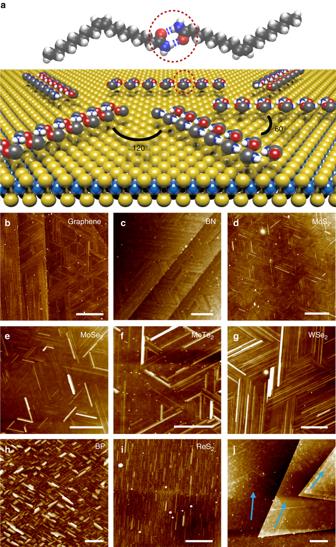Fig. 1 Self-assembly of oleamide on various 2D atomic crystals.aSchematic representation of oleamide self-assembly on 2D atomic crystals along specific orientations. For clarity, only the amide groups are displayed and the alkyl chains of oleamide are not shown except for the topmost oleamide dimer which shows the complete molecular structures. Hydrogen bonds are indicated withblue dashedlines.White,gray,blueandredballs represent H, C, N and O atoms, respectively.b–iAFM images of oleamide nanoribbons on graphene,h-BN, MoS2, MoSe2, MoTe2, WSe2,blackphosphorus (BP) and ReS2, respectively.jNanoribbons on CVD-grown multilayer MoS2.Blue arrowsrepresent the orientations of nanoribbons on varied layers. Allscale barsare 500 nm, except for that incwhich is 200 nm Probing the crystallographic orientation of two-dimensional (2D) materials is essential to understand and engineer their properties. However, the nondestructive identification of the lattice orientations of various 2D materials remains a challenge due to their very thin nature. Here, we identify the crystallographic structures of various 2D atomic crystals using molecules as probes by utilizing orientation-dependent molecule–substrate interactions. We discover that the periodic atomic packing of 2D materials guides oleamide molecules to assemble into quasi-one-dimensional nanoribbons with specific alignments which precisely indicate the lattice orientations of the underlying materials. Using oleamide molecules as probes, we successfully identify the crystallographic orientations of ~12 different 2D materials without degrading their intrinsic properties. Our findings allow for the nondestructive identification of the lattice structure of various 2D atomic crystals and shed light on the functionalization of these 2D materials with supramolecular assembly. Two-dimensional (2D) atomic crystals, endowed with unique ultrathin planar and well-ordered atomic structures, have shown a broad range of attractive properties, which are dramatically different from their bulk counterparts [1] , [2] . Among these properties, electrical transport [3] , [4] , thermal conductance [5] , [6] , piezoelectric characteristics [7] , optical properties [3] and so on are significantly dependent on their 2D crystallographic orientations, especially for those with in-plane anisotropic structures such as black phosphorus [3] and ReS 2 [4] . Besides these intrinsic properties, modulating the properties of 2D atomic crystals by strain, stacking and size-confinement is also highly dependent on their pristine lattice orientations as indicated by various theoretical and experimental studies [8] , [9] , [10] . Therefore, probing the crystallographic orientation of these materials is essential for understanding and controllably tuning their properties in an expanding array of 2D atomic materials. The most straightforward characterization is to directly image the atomic structure of 2D materials with scanning transmission electron microscope (STEM) [11] or scanning tunneling microscope (STM) [12] . However, the acquisition of atomically resolved images by both STEM and STM has critical requirements on sample preparation, equipment and imaging skills, which makes these approaches very expensive and low throughput. More importantly, the imaged samples are located on specialized substrates such as transmission electron microscope grids or conducting substrates, which hinders their further applications. Recently, orientation-dependent intensities of second harmonic generation (SHG) and polarized Raman spectroscopy have been observed in several 2D atomic crystals, providing an alternative approach for identifying lattice orientation of several 2D materials, such as odd-layered BN [13] , MoS 2 [14] , WS 2 [15] and GaSe [16] by SHG and black phosphorus [17] and ReS 2 (ReSe 2 ) [18] , [19] , [20] by Raman spectroscopy. Unfortunately, these spectroscopic approaches have strict requirements on the symmetry and structures of the materials and thus cannot be adapted to identify the crystallographic orientations of a large variety of 2D materials. A universal and nondestructive approach for rapidly probing the lattice orientation of various 2D atomic crystals is therefore crucial to advance the field of 2D atomic crystals. Organizing molecules into geometric order on surfaces has attracted extensive interest for constructing nano-devices and nanostructured materials using bottom-up approaches [21] . It is well-accepted that molecule–substrate interactions significantly affect the adsorption of single molecules on solid surfaces and thus can guide the orientation of molecules [22] . Much effort has been made to investigate the effects of substrate surface structure on the assembly of molecules [23] , [24] . However, whether the geometry of the resulting supramolecular structures can reveal the atomic structures of the substrate has not been explored. We expect that periodic atomic arrangements of 2D atomic crystals result in periodic molecule–substrate interactions in the 2D plane and thus provide a unique landscape for aligning molecules. Proceeding from this point, we explore the self-assembly of molecules on 2D atomic crystals from both experimental and theoretical aspects and successfully develop a universal, simple and nondestructive approach to identify the lattice structures of various 2D atomic crystals using molecules as probes. Orientation-selected assembly of oleamide molecules on 2D atomic crystals The well-ordered assembly of various molecules has been explored mainly on the surfaces of metals and graphite by STM imaging [22] . Among these molecules, here, we choose oleamide as the probe to identify the lattice orientations of 2D atomic crystals as these molecules can form anisotropic quasi-one-dimensional (1D) structures driven by intermolecular hydrogen bonds on highly orientated pyrolytic graphite [25] , [26] , which is highly desirable for indicating the lattice orientation of the substrates. The assembly process of oleamide onto 2D atomic crystals simply involves two steps: spin-coat a drop of dilute oleamide solution in chloroform onto 2D materials and then anneal the samples at 60 o C for 30 min (see Methods for experimental details). After the assembly, dense nanoribbons (500 ± 200 nm, 50 ± 20 nm and 5 ± 4 nm in length, width and height, respectively, as shown in Supplementary Fig. 1 ) were observed on various hexagonal 2D atomic crystals such as mechanically exfoliated graphene, h -BN, MoS 2 , MoSe 2 , MoTe 2 , WS 2 , WSe 2 , NbSe 2 , TaS 2 and so on (Fig. 1b–g and Supplementary Fig. 2), and these nanoribbons aligned along three directions with rotations of ~120 o (Supplementary Fig. 3 ) as schematically illustrated in Fig. 1a over a large area (Supplementary Figs. 4 and 5 ). In addition to these hexagonal crystals, nanoribbons on black phosphorus with tetragonal symmetry and ReS 2 with distorted 1T structure also displayed specific orientations along two and one directions, respectively (Fig. 1h, i ). We ruled out the possible formation of oleamide nanoribbons in solution through dynamic light scattering (DLS) measurements (Supplementary Fig. 6 ) and a control experiment on the self-assembly of 5, 10, 15, 20-tetraphenyl-21H, 23H-porphine cobalt (II) (CoTPP) on MoS 2 (Supplementary Figs. 6 and 7 ), and therefore, confirmed that oleamide nanoribbons were formed on the surface of 2D materials instead of in solution. The dramatically different orientations of oleamide nanoribbons on 2D atomic crystals with varied crystallographic structures suggest that the alignment of nanoribbons is very likely to be guided by the atomic structures of the underlying substrates. Fig. 1 Self-assembly of oleamide on various 2D atomic crystals. a Schematic representation of oleamide self-assembly on 2D atomic crystals along specific orientations. For clarity, only the amide groups are displayed and the alkyl chains of oleamide are not shown except for the topmost oleamide dimer which shows the complete molecular structures. Hydrogen bonds are indicated with blue dashed lines. White , gray , blue and red balls represent H, C, N and O atoms, respectively. b – i AFM images of oleamide nanoribbons on graphene, h -BN, MoS 2 , MoSe 2 , MoTe 2 , WSe 2 , black phosphorus (BP) and ReS 2 , respectively. j Nanoribbons on CVD-grown multilayer MoS 2 . Blue arrows represent the orientations of nanoribbons on varied layers. All scale bars are 500 nm, except for that in c which is 200 nm Full size image Orientation-correlations between oleamide nanoribbons and 2D materials To correlate the orientations of the oleamide nanoribbons with the lattice structure of 2D atomic crystals, we characterized several 2D atomic crystals with oleamide assembly by combining STEM, SHG and polarized Raman spectroscopy. We first recorded the geometry of MoS 2 flakes with oleamide assembly by atomic force microscope (AFM) and then selectively transferred the same MoS 2 flake to a holey carbon grid for atomically resolved STEM imaging (Fig. 2a, b , see Supplementary Methods for experimental details). The correlation between the orientations of the nanoribbons and the MoS 2 atomic structures can be accurately affirmed by overlapping the geometric images taken by AFM and STEM (Supplementary Fig. 8a, b ) and the results confirmed that oleamide nanoribbons oriented along the zigzag directions of MoS 2 lattice (see Supplementary Note 1 for more details). Besides STEM imaging, SHG was also utilized to characterize the lattice orientations of MoS 2 with oleamide nanoribbons. The angle-resolved SHG intensity measured on monolayer MoS 2 (Fig. 2c ) with oleamide nanoribbons shows a clear six-petal pattern and the maximum petal direction points to the armchair lattice orientations of MoS 2 (Fig. 2d ) [14] . Hence, the zigzag lattice orientations of the MoS 2 monolayer are determined by rotating the armchair directions by 30 o , which are exactly the same as the orientations of the nanoribbons shown in Fig. 2c , again, confirming that oleamide nanoribbons align along the zigzag orientations of MoS 2 . Besides MoS 2 , we conducted SHG measurement on WSe 2 with oleamide nanoribbons and obtained the same conclusion (Supplementary Fig. 9 ). Fig. 2 Correlations between the orientations of oleamide nanoribbons and the lattice of underlying 2D materials. a , b AFM image and Fourier filtered STEM image of the same few-layer MoS 2 flake with oleamide nanoribbons. Inset Schematic representation of top view of MoS 2 atomic structures. Red arrows correspond to the orientations of nanoribbons on this flake. c , d AFM image and polarization angle-dependent SHG intensity plot of the same monolayer MoS 2 flake with oleamide nanoribbons. The black dashed arrows indicate the zigzag directions of this MoS 2 flakes determined by SHG and the red arrows correspond to the orientations of nanoribbons on this flake. e , f AFM image and Fourier filtered STEM image of the same multilayer black phosphorus flake with oleamide nanoribbons. Inset Schematic representation of top view of the atomic structure of black phosphorus. Red arrows correspond to the orientations of nanoribbons. The black dashed arrow indicates the armchair direction of this flake. g , h AFM image and angle-dependent polarized Raman intensity plot of the same multilayer black phosphorus flake with oleamide nanoribbons. The black dashed arrow indicates the armchair direction of this flake determined by Raman measurements and the red arrows indicate the orientations of the nanoribbons on this flake. Scale bars for a , c , e and g are 500 nm and for b , f are 1 nm Full size image Besides hexagonal 2D materials with threefold symmetry, we also explored the correlations between the nanoribbon orientations and the lattice structures of 2D black phosphorus with tetragonal symmetry and ReS 2 with triclinic symmetry (Fig. 2e and Supplementary Fig. 10c ) with atomically resolved STEM and angle-resolved polarized Raman spectroscopy. Following the similar STEM imaging process of MoS 2 , the armchair orientation of black phosphorus is determined to be along the bisector of the nanoribbon directions, with rotations of 33 o to each nanoribbon orientations (Fig. 2e, f ). Polarized Raman spectroscopy measurements on 2D black phosphorus with oleamide nanoribbons also revealed the same relationship between the orientations of nanoribbons and the armchair direction of black phosphorus (Fig. 2g, h ) [27] . Likewise, the nanoribbons assembled on ReS 2 were verified to be aligned along the direction of Re chains (zigzag lattice structure) using angle-resolved polarized Raman spectroscopy (Supplementary Fig. 10 ) [18] . So far, we have demonstrated that the preferred orientations of oleamide nanoribbons can be well-correlated with the lattice structure of 2D atomic crystals experimentally. Theoretical calculations on the surface-templated assembly of oleamide Next, we investigated the origins for the preferred orientations of oleamide nanoribbons on 2D atomic crystals from theoretical aspects. The orientation of an oleamide molecule on 2D atomic crystals is dictated by the van der Waals interactions between adsorbate and substrate. So we first calculated the rotation potential energy curve of a single oleamide molecule on monolayer MoS 2 with only Grimme’s D3 dispersion parameters (Supplementary Fig. 11 ) and the adsorption energy of a single oleamide molecule aligned along either zigzag or armchair direction of monolayer MoS 2 by the DFT-D3 method [28] (see Supplementary Methods for calculation details). For each alignment, we performed 2D potential energy surface (PES) scan to ascertain the most favorable adsorption position by accounting for only dispersion interactions between oleamide and MoS 2 . The 2D PES for zigzag aligned oleamide and its 1D projection along the x (zigzag) and y (armchair) directions respectively have been shown in Fig. 3a, b . The energy valleys in Fig. 3a exhibit the same hexagonal symmetry as the underlying lattice of MoS 2 . Our DFT-D3 calculations of the adsorption energy show that the zigzag aligned oleamide is favored by 0.11 eV as compared to the armchair aligned one. Because the interactions between oleamide molecules and the surface are stronger than the intermolecular interactions between oleamide molecules [26] , the surface lattice will template the formation of nanostructures that cannot be formed in solution [25] (Supplementary Fig. 6 ). Thus the adsorbate-substrate interactions dictate the assembly of oleamide molecules on the surface of 2D atomic crystals and the tendency to achieve maximum H-bonding between –C=O and -NH 2 groups of adjacent molecules servers as secondary interactions [26] . Based on the thermodynamically most stable adsorption position of individual zigzag aligned oleamide, we constructed the assembly pattern of oleamide molecules on MoS 2 (Fig. 3c ). In this pattern, oleamide molecules not only form H-bonded dimers in a head-to-head configuration but also H-bonded nanoribbons in a side-by-side configuration. The orientations of nanoribbons are along the zigzag lattice directions of the underlying MoS 2 , as also clearly seen from Fig. 3a . Our calculations also confirm that oleamide molecules form H-bonded nanoribbons on other hexagonal 2D atomic crystals including graphene, BN, MoSe 2 , MoTe 2 and WS 2 , along the zigzag lattice directions (Supplementary Fig. 12 and Supplementary Note 2 ). The first molecular layer of nanoribbons will in turn template the second layer assembly, and so on. The rotation and 2D PES scan showed that the second layer oleamide molecules and all layers above align along the same direction as the first molecular layer and stack right on top of the molecules in the bottom layers (Supplementary Fig. 13 and Supplementary Note 3 ). Similar calculations can be performed on other 2D atomic crystals to reveal their respective preferred adsorption directions. Fig. 3 Theoretical calculations of oleamide assembly on monolayer MoS 2 . a 2D potential energy surface (PES) of a single oleamide molecule adsorbed on MoS 2 , with one oleamide subchain aligned along the zigzag lattice direction of substrate. The 2D PES exhibits the same hexagonal symmetry as the underlying lattice of MoS 2 . The energy valleys in blue represent the most stable adsorption positions for zigzag aligned oleamide molecules. b 1D projection along the x (zigzag) and y (armchair) directions of the same 2D PES in a . c Assembly of oleamide molecules on MoS 2 . Each oleamide molecule is adsorbed onto the MoS 2 surface at the thermodynamically most stable position, as indicated by the energy valley of the 2D PES in a . The red arrow on the left indicates the orientation of the nanoribbon, which is exactly the zigzag lattice direction of MoS 2 . The color code of the atoms is Mo: light blue , S: yellow , C: gray , H: white , O: red , and N: dark blue , respectively Full size image Universal and nondestructive identification with oleamide As both experimental and theoretical studies have confirmed that oleamide molecules can be used to probe the lattice orientations of various 2D atomic crystals, we further demonstrated the applications of this approach to identifying the edge orientations, grain domain and stacking rotations, which all significantly affect the intrinsic properties of these materials. Besides mechanically exfoliated 2D materials, well-aligned oleamide nanoribbons were also observed on chemical vapor deposition (CVD)-grown MoS 2 regardless of the number of layers (Fig. 1j ). With this approach, we identified that the edges of CVD-grown MoS 2 flakes were along zigzag directions as the nanoribbons orientated parallel to the edges of the triangular CVD-grown MoS 2 flakes, which is consistent with the STEM imaging (Fig. 1j and Supplementary Fig. 14 ). In addition to the as-grown edges, the MoS 2 edges created by oxygen etching were also identified to be along zigzag directions of MoS 2 lattice by using oleamide nanoribbons as probes (Supplementary Fig. 15a and Supplementary Note 4 ). Moreover, the grain domain in polycrystalline CVD-grown MoS 2 and the interlayer rotation angles in multilayer MoS 2 can also be easily identified with this approach (Supplementary Fig. 15b, c and Fig. 1j ). Therefore, this approach is universal in determining the lattice orientations of various 2D atomic crystals, regardless of the chemical compositions, preparation methods and geometry. Besides being universal in identifying different kinds of 2D atomic crystals, the most prominent advantages of our identification approach is that it is simple and nondestructive. This identification process is very simple as only conventional AFM imaging is involved to observe the orientation of oleamide nanoribbons. This process can be further simplified to directly image the orientation of the oleamide assembly with an optical microscope as some of the nanoribbons can grow up to micrometer scale (Fig. 4b, c ) as the result of molecule transfer from smaller nanoribbons with higher chemical potential to bigger ones with lower chemical potential, similar to the Ostwald ripening of crystals in a liquid phase (Fig. 4a ) [29] , [30] . More importantly, this approach is nondestructive as the melting point of oleamide is relatively low (~75 o C) and thus can desorb from the surface of the 2D atomic crystals during storage under ambient conditions (Supplementary Fig. 16 ). To speed up the desorption, we annealed the MoS 2 samples with oleamide assembly in vacuum at 300 o C for 1 h and observed that all the nanoribbons vanished (Figs. 4d, e ) without inducing obvious peak position shift in photoluminescence (PL) and Raman spectra (Fig. 4f , Supplementary Fig. 17 and Supplementary Note 5 ) and the surface roughness of the MoS 2 flakes was identical to the pristine value after the removal (0.264 nm (before) and 0.269 nm (after)). To further rule out the possible degradation on the intrinsic properties of MoS 2 by the identification process, we fabricated back-gated field effect transistors on both pristine and identified monolayer MoS 2 (Supplementary Fig. 18 ) and compared their electrical performances. The averaged mobility of monolayer CVD-grown MoS 2 flakes that underwent oleamide assembly and removal is ~ 8 cm 2 V −1 s −1 , similar to the value obtained from their pristine counterparts (Fig. 4g ), indicating that the intrinsic properties of underlying 2D atomic crystals can be well preserved throughout the whole processes. Fig. 4 Optical visualization and nondestructive removal of oleamide nanoribbons. 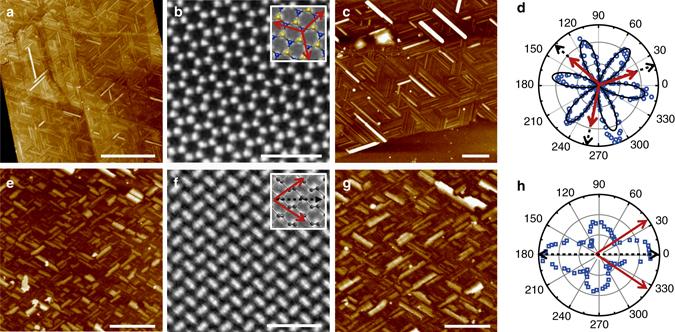Fig. 2 Correlations between the orientations of oleamide nanoribbons and the lattice of underlying 2D materials.a,bAFM image and Fourier filtered STEM image of the same few-layer MoS2flake with oleamide nanoribbons.InsetSchematic representation of top view of MoS2atomic structures.Red arrowscorrespond to the orientations of nanoribbons on this flake.c,dAFM image and polarization angle-dependent SHG intensity plot of the same monolayer MoS2flake with oleamide nanoribbons. Theblack dashedarrows indicate the zigzag directions of this MoS2flakes determined by SHG and thered arrowscorrespond to the orientations of nanoribbons on this flake.e,fAFM image and Fourier filtered STEM image of the same multilayer black phosphorus flake with oleamide nanoribbons.InsetSchematic representation of top view of the atomic structure of black phosphorus.Red arrowscorrespond to the orientations of nanoribbons. Theblack dashed arrowindicates the armchair direction of this flake.g,hAFM image and angle-dependent polarized Raman intensity plot of the same multilayer black phosphorus flake with oleamide nanoribbons. Theblack dashed arrowindicates the armchair direction of this flake determined by Raman measurements and thered arrowsindicate the orientations of the nanoribbons on this flake.Scale barsfora,c,eandgare 500 nm and forb,fare 1 nm a , Schematic for the evolution of nanoribbons driven by chemical potential. Small nanoribbons shrink while the large ones grow up. b , c AFM images of oleamide nanoribbons on a few-layer MoS 2 flake after 1 h and 8 days under ambient condition, respectively. Scale bar , 1 µm. Inset Optical images. Scale bar , 2 μm. d , e AFM images of a monolayer MoS 2 flake with oleamide nanoribbons before and after annealing in vacuum at 300 o C for 1 h, respectively. Scale bars , 500 nm. f PL spectra collected from the same monolayer MoS 2 : pristine ( black ), after oleamide self-assembly ( red ), and after the removal of nanoribbons ( blue ). g Typical I ds - V gs curve for CVD-grown monolayer MoS 2 flakes after the removal of nanoribbons ( V ds = 1 V). Inset The averaged mobility of pristine ( blue ) and identified MoS 2 after the removal of nanoribbons ( red ) Full size image In summary, we explore the self-assembly of molecules on various 2D atomic crystals by using oleamide molecules as an example both from experimental and theoretical aspects. We show that the periodic atomic arrangements of these materials can guide the assembly of molecules into well-ordered supramolecular structures and correlate the orientations of the oleamide assembly with the lattice structure of the underlying 2D atomic crystals. With self-assembled oleamide nanoribbons as probes, the crystallographic orientations, grain boundaries and stacking configurations of a large variety of 2D atomic crystals regardless of preparation methods and geometry can be easily identified. More importantly, this approach is nondestructive as confirmed by both spectroscopic and electrical measurements, which enables further applications of the identified materials. By using molecules as probes, we open up a new way for simple and nondestructive identification of lattice structures of various substrates especially for 2D atomic crystals, which greatly facilitates both fundamental and application studies of these emerging materials. Preparation of 2D materials The 2D atomic crystals were obtained by mechanical exfoliation of bulk crystals purchased from 2D Semiconductors on SiO 2 /Si substrates with Scotch tape, followed by annealing in vacuum at 320 o C for 30 min to remove residual tape (290 o C for ReS 2 ) before the assembly of oleamide. CVD-grown MoS 2 flakes were obtained using electrochemical oxidized Mo foils as precursors and the growth was carried out at 650−800 o C [31] . 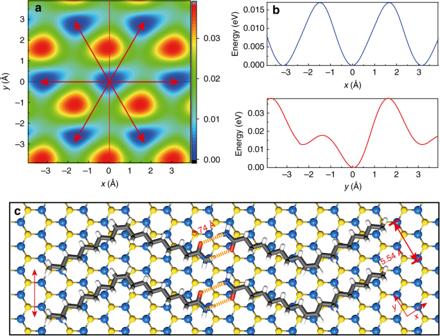Fig. 3 Theoretical calculations of oleamide assembly on monolayer MoS2.a2D potential energy surface (PES) of a single oleamide molecule adsorbed on MoS2, with one oleamide subchain aligned along the zigzag lattice direction of substrate. The 2D PES exhibits the same hexagonal symmetry as the underlying lattice of MoS2. The energy valleys inbluerepresent the most stable adsorption positions for zigzag aligned oleamide molecules.b1D projection along thex(zigzag) andy(armchair) directions of the same 2D PES ina.cAssembly of oleamide molecules on MoS2. Each oleamide molecule is adsorbed onto the MoS2surface at the thermodynamically most stable position, as indicated by the energy valley of the 2D PES ina. Thered arrowon theleftindicates the orientation of the nanoribbon, which is exactly the zigzag lattice direction of MoS2. The color code of the atoms is Mo:light blue, S:yellow, C:gray, H:white, O:red, and N:dark blue, respectively 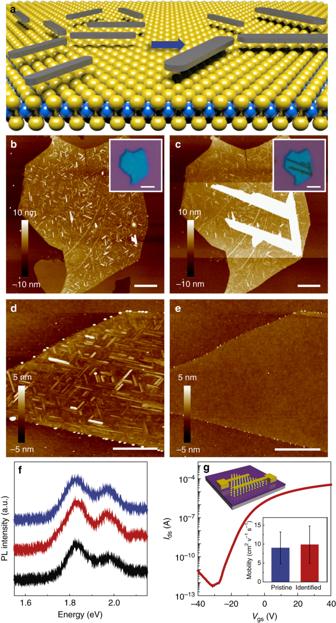Fig. 4 Optical visualization and nondestructive removal of oleamide nanoribbons.a, Schematic for the evolution of nanoribbons driven by chemical potential. Small nanoribbons shrink while the large ones grow up.b,cAFM images of oleamide nanoribbons on a few-layer MoS2flake after 1 h and 8 days under ambient condition, respectively.Scale bar, 1 µm.InsetOptical images.Scale bar, 2 μm.d,eAFM images of a monolayer MoS2flake with oleamide nanoribbons before and after annealing in vacuum at 300oC for 1 h, respectively.Scale bars, 500 nm.fPL spectra collected from the same monolayer MoS2: pristine (black), after oleamide self-assembly (red), and after the removal of nanoribbons (blue).gTypicalIds-Vgscurve for CVD-grown monolayer MoS2flakes after the removal of nanoribbons (Vds= 1 V).InsetThe averaged mobility of pristine (blue) and identified MoS2after the removal of nanoribbons (red) Self-assembly of oleamide on 2D materials The assembly of oleamide was performed by spin coating 7 µL dilute solution (1.65 mmol L −1 ) of oleamide (Sigma-Aldrich, 99%) in chloroform (Alfa Aesar, 99%) on 2D materials at 2400 r.p.m. for 1 min, followed by baking at 60 o C for 30 min, except for black phosphorus. To prevent the oxidation of black phosphorus, the mechanical exfoliation of black phosphorus and the spin coating of oleamide were conducted in a glove box without baking. Characterization of nanoribbon/2D materials AFM images were captured with Bruker Dimension Icon in ScanAsyst mode. The optical images were taken with an Olympus BX 51 M microscope. Raman and PL spectra were collected with Horiba-Jobin-Yvon Raman system under 532 nm laser excitation with a power of 2 mW. The Si peak at 520.7 cm −1 was used for calibration. SHG measurements were conducted under an 820 nm femtosecond laser with excitation power of 0.4 mW (Spectra-Physics® Inspire™ ultrafast OPO system with tunable wavelength of 345–2500 nm, pulse duration of 100 fs and repetition rate of 80 MHz). Linearly polarized excitation light was focused on the sample by an Nikon objective (100X, N.A. = 0.95). SHG signal was detected with a spectrometer (Princeton Instruments, Acton SpectraPro® SP2500 PYLON). Atomically resolved high-angle annular dark-field STEM images were taken with an ARM-200CF (JEOL) transmission electron microscope operated at 200 kV and equipped with double spherical aberration (Cs) correctors. The attainable resolution of the probe defined by the objective pre-field is 78 picometers. Data availability The data that support the findings of this study are available from the corresponding authors on request.